Design amphiphilic dipolar π-systems for stimuli-responsive luminescent materials using metastable states π-Conjugated compounds that exhibit tunable luminescence in the solid state under external mechanical stimuli have potential applications in sensors and imaging devices. However, no rational designs have been proposed that impart these mechano-responsive luminescent properties to π-conjugated compounds. Here we demonstrate a strategy for mechano-responsive luminescent materials by imparting amphiphilic and dipolar characteristics to a luminescent π-conjugated system. The oligo( p -phenylenevinylene) luminophore with a didodecylamino group at one end and a tri(ethylene glycol) ester group at the other end yields segregated solid structures by separately aggregating its hydrophobic and hydrophilic moieties. The segregated structures force the molecules to align in the same direction, thereby generating a conflict between the side-chain aggregation and dipolar stabilization of the π-system. Consequently, these metastable solid structures can be transformed through mechanical stimulation to a more stable structure, from a π–π stacked aggregate to a liquid crystal and further to a crystalline phase with variable luminescence. Organic, π-conjugated materials that exhibit tunable luminescent properties in the solid state under external stimuli can be applied in optical devices, displays, fluorescent probes and sensors [1] , [2] , [3] , [4] . Recently, luminescent materials that are responsive to mechanical stimuli have attracted considerable attention because they have the unique ability to tune their molecular, physical or chemical properties via macroscopic stimulation [5] , [6] , [7] , [8] . Several mechanistic explanations for the mechanically stimulated changes in the colour of the luminescence have been proposed: a phase transformation of the solid structure [9] , [10] , [11] , [12] , [13] , [14] , [15] , [16] , excimer formation or dissolution [17] , [18] , [19] and mechanical stress-induced chemical changes [20] , [21] . However, the development of new materials with luminescent mechanochromism still depends heavily on serendipitous discovery or random screening; studies based on rationally designed luminophoric compounds and sensitivity to mechanical stimuli remains rare. One possible strategy for designing stimulus-sensitive materials involves generating metastable, kinetically trapped states in the luminophoric compounds with emission properties that are sensitive to the surrounding environment. When a mechanical stimulus converts the metastable state to a more thermodynamically stable solid state with new emission properties, a mechano-responsive change occurs in the compound’s luminescence. Here we report a new mechanochromic material created using a molecular-level design according to the aforementioned strategy. To obtain metastable, self-assembled states, we imparted amphiphilic and dipolar characteristics to a luminescent π-conjugated system. The π-conjugated molecule can adopt a segregated solid structure by aggregating its hydrophobic and hydrophilic moieties separately ( Fig. 1a ) [22] , [23] , [24] . The segregated structure would force the molecules to align in the same direction, thereby generating a conflict between the side-chain aggregation and dipolar stabilization of the core [22] . Consequently, this designed metastable aggregate structure could be easily transformed to more stable structures with variable luminescence. 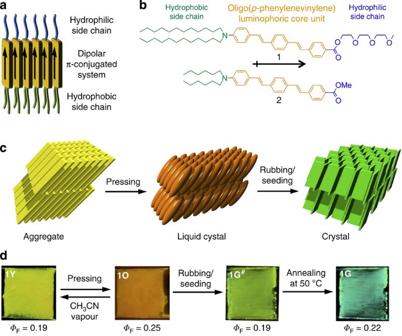Figure 1: Stimuli-responsive change in luminescence and phase of1. (a) Schematic representation of the segregated packing structure of amphiphilic dipolar molecule. (b) Molecular structure of amphiphilic dipolar luminophore1and reference compound2. (c) Schematic representation of stimuli-responsive phase transition of1. (d) Photographs of a thin film of1(~0.8 × 0.8 cm2) showing stimuli-responsive change in the luminescence under UV (365 nm) irradiation. Figure 1: Stimuli-responsive change in luminescence and phase of 1. ( a ) Schematic representation of the segregated packing structure of amphiphilic dipolar molecule. ( b ) Molecular structure of amphiphilic dipolar luminophore 1 and reference compound 2 . ( c ) Schematic representation of stimuli-responsive phase transition of 1 . ( d ) Photographs of a thin film of 1 (~0.8 × 0.8 cm 2 ) showing stimuli-responsive change in the luminescence under UV (365 nm) irradiation. Full size image Molecular design In this study, molecule 1 was designed to exhibit various stimuli-responsive properties ( Fig. 1b ). Compound 1 contains three different segments: a polarized luminophoric core of oligo( p -phenylenevinylene) [25] , [26] , [27] , an electron-donating amino group with hydrophobic dodecyl chains (C 12 H 25 ) and an electron-withdrawing ester group with a hydrophilic tri(ethylene glycol) (TEG) chain. The amino and ester groups render the core portion moderately polar ( μ =6.8 D based on a density functional theory (DFT) calculation) and impart intramolecular charge–transfer abilities to the excitation state because the destabilized highest occupied molecular orbital (HOMO) is more localized around the amino group, whereas the stabilized lowest unoccupied molecular orbital (LUMO) remains more localized around the ester group ( Fig. 2a ). In solution, 1 exhibits a notable solvatochromic photoluminescence shift from blue to red when the solvent polarity changes from ε (dielectric constant)=1.88 (hexane, λ em-max =488 nm, Φ F =0.79) to ε =37.5 (acetonitrile, λ em-max =685 nm, Φ F =0.23) ( Fig. 2b ), whereas the absorption spectra remain unchanged ( Supplementary Fig. 1 and Supplementary Table 1 ). These results indicate that 1 has excited-state energy levels associated with intramolecular charge transfers. Therefore, in the condensed state, the photoemission properties of 1 should also be sensitive to the microenvironment and to molecular arrangements. 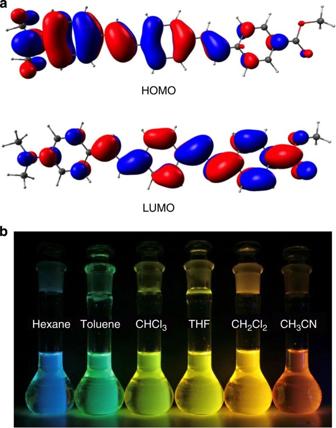Figure 2: Molecular orbitals and photoluminescence colors of dipolar oligo(p-phenylenevinylene) in various solvents. (a) Molecular orbitals (top: HOMO and bottom: LUMO) of a model dipolar oligo(p-phenylenevinylene) molecule (asymmetrically substituted with -COOCH3and -N(CH3)2groups) obtained by DFT calculation at B3LYP/6-311++G(d,p). (b) Photographs of the solutions of1in various organic solvents (from left to right: hexane, toluene, chloroform, tetrahydrofuran, dichloromethane and acetonitrile) under UV (365 nm) irradiation. Figure 2: Molecular orbitals and photoluminescence colors of dipolar oligo( p -phenylenevinylene) in various solvents. ( a ) Molecular orbitals (top: HOMO and bottom: LUMO) of a model dipolar oligo( p -phenylenevinylene) molecule (asymmetrically substituted with -COOCH 3 and -N(CH 3 ) 2 groups) obtained by DFT calculation at B3LYP/6-311++G(d,p). ( b ) Photographs of the solutions of 1 in various organic solvents (from left to right: hexane, toluene, chloroform, tetrahydrofuran, dichloromethane and acetonitrile) under UV (365 nm) irradiation. Full size image Mechanochromic luminescence Compound 1 initially exhibited yellow photoluminescence after being drop cast onto a glass substrate; after the sample was pressed, the luminescence became orange. An anisotropic mechanical stimulus (rubbing) applied to the material’s surface triggered a phase change to a crystalline material with green photoluminescence. Even when the rubbing area was small, the phase conversion spontaneously propagated across the entire sample area. An analysis of the structural and optical properties of the phases revealed that the variable luminescence originates from the alteration of the intermolecular interaction and the conformation of the π-conjugated luminophores upon the mechanical induction of phase transitions from aggregate to mesophase to crystal ( Fig. 1c ). Figure 1d outlines the stimuli-responsive luminescent colour change of 1 , whereas Fig. 3 illustrates optical microscopy (OM), polarized OM (POM) and fluorescence microscopy images typical of each phase. We obtained a thin film ( 1Y ) that exhibited yellow photoluminescence (fluorescence quantum yield, Φ F =0.19) after casting aqueous acetonitrile solutions of 1 . OM and POM images showed the formation of birefringent, sheet-like micro objects (microsheets; Fig. 3a,b ). After being pressed or gently ground, 1Y became a waxy, fluidic and highly birefringent mesophase ( 1O ; Fig. 3c,d ). The 1Y → 1O phase transition was accompanied by a change in the photoluminescence from yellow to orange ( Φ F =0.25) ( Supplementary Movie 1 ). The mesomorphic phase 1O could be reverted to 1Y by exposure to acetonitrile vapour. To our surprise, vigorous grinding of 1O triggered a crystallization and a further change in the photoluminescence to yellowish green ( 1G # , Φ F =0.19). Thermal annealing of 1G # at 50 °C generated a bluish-green emission ( 1G , Φ F =0.22; Fig. 3e,f ). Because POM ( Supplementary Fig. 2a ), differential scanning calorimetry (DSC; Supplementary Fig. 2b ), powder X-ray diffraction (PXRD; Supplementary Fig. 3 ) and ultraviolet/visible (UV/Vis) studies ( Supplementary Fig. 4 ) indicated that 1G # was a less crystalline form of 1G , we focused on 1Y , 1O and 1G during the subsequent structural studies. 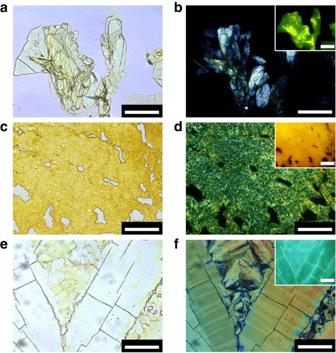Figure 3: Optical micrographs showing mechanically induced phase transition of1. (a,b) Optical micrograph (a) and polarized optical micrograph (b) of microsheets of1Y. (c,d) Optical micrograph (c) and polarized optical micrograph (d) of mesophase of1O. (e,f) Optical micrograph (e) and polarized optical micrograph (f) of crystallites of1G. Scale bars, 100 μm in all the images. Insets inb,dandfare the corresponding fluorescence micrographs of each phase. Figure 3: Optical micrographs showing mechanically induced phase transition of 1. ( a , b ) Optical micrograph ( a ) and polarized optical micrograph ( b ) of microsheets of 1Y . ( c , d ) Optical micrograph ( c ) and polarized optical micrograph ( d ) of mesophase of 1O . ( e , f ) Optical micrograph ( e ) and polarized optical micrograph ( f ) of crystallites of 1G . Scale bars, 100 μm in all the images. Insets in b , d and f are the corresponding fluorescence micrographs of each phase. Full size image Thermal properties The DSC analyses revealed that 1Y , 1O and 1G exhibit different thermal stabilities ( Fig. 4 ). A heated scan of 1Y revealed a broad endothermic peak at ~37 °C (Δ H =11.5 kcal mol –1 ). POM observations showed that this peak was caused by the thermal transition of 1Y to 1O (see below). The resultant 1O became the isotropic phase ( Iso ) at 47 °C (Δ H =1.4 kcal mol –1 ); this result is consistent with the clearing temperature of the mechanically induced 1O (47 °C, Δ H =4.4 kcal mol –1 ). These results indicate that the molecular packings of mechanically and thermally induced 1O are potentially identical. In contrast, the crystalline phase 1G transformed into Iso at 54 °C (Δ H =12.7 kcal mol –1 ), achieving the most stable molecular packing. All isotropic phases exhibited two exothermic transitions at ~44 °C and 38 °C, respectively, upon cooling, without the hysteresis observed in the pre-melt phases. The POM observations indicated that the upper transition corresponded to the thermal generation of mesomorphic 1O , whereas the lower transition was accompanied by no apparent change in the POM textures as well as emission properties. Taking into account a small change of interlayer distance ( d =32.6→34.2 Å, see the next section) and a small enthalpy change (–0.5 kcal mol –1 ) upon the lower transition, a minor structural change that is associated with the molecular tilt might occur in 1O at 38 °C upon cooling. 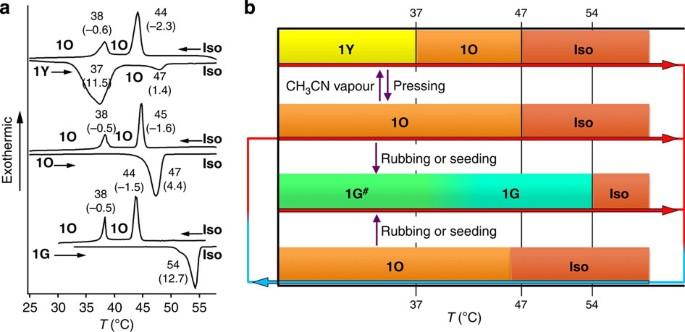Figure 4: Thermal behaviour of1. (a) DSC traces (2 °C min−1) of1Y,1Oand1Gwith the phase-transition temperatures in °C and associated enthalpy changes (in brackets) in kcal mol–1. (b) Phase-transition behaviour of1. Heating and cooling procedures are indicated by red and blue arrows, respectively. Figure 4: Thermal behaviour of 1 . ( a ) DSC traces (2 °C min −1 ) of 1Y , 1O and 1G with the phase-transition temperatures in °C and associated enthalpy changes (in brackets) in kcal mol –1 . ( b ) Phase-transition behaviour of 1 . Heating and cooling procedures are indicated by red and blue arrows, respectively. Full size image Molecular packing The PXRD measurements of 1 ’s three distinct phases indicated that the mechanical stimuli induced explicit transformations in the material’s molecular packing. The PXRD pattern of 1Y was characterized by numerous reflections with a reciprocal spacing ratio 1:2:3:4:6:7 for 42.7 Å ( Fig. 5a ). Atomic force microscopy (AFM) observation of the surface of the microsheets of 1Y visualized the elementary layers with thicknesses of ~4 nm ( Fig. 5b ), which is consistent with the PXRD results. The emergence of up to (007) reflections demonstrates that a long-range ordered, multilamellar structure was formed. Because the molecular length of 1 was ~42 Å, the observed layer spacing indicates that a bilayer structure was formed with a considerable molecular tilt and interdigitated TEG side chains ( Fig. 5e ). In the wide-angle region, the reflection corresponding to the crystalline alkyl chain was observed at d =4.3 Å, along with other small reflections that could be derived from the in-plane molecular ordering within the lamellae. 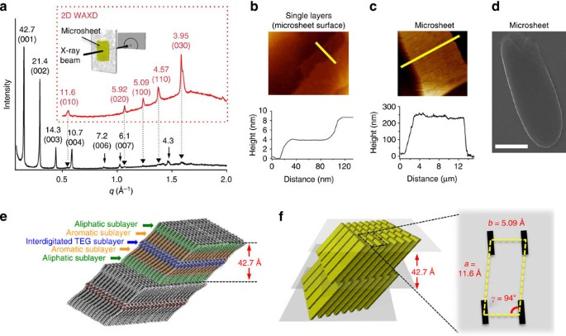Figure 5: Analysis of packing structures of1Y. (a) PXRD patterns of1Ywith majord-spacings in Å. Small diffractions derived from the in-plane molecular ordering are indicated by black triangles. Inset (surrounded by red dotted square): Schematic representation for the experimental setup of transmission mode 2D-WAXD of1Ymicrosheets deposited on 0.03-mm thickness glass substrate using synchrotron radiation and the observed diffraction profile. (b) AFM image of the surface of1Ymicrosheet and a cross-sectional analysis along to the yellow line. (c) AFM image of the surface of1Ymicrosheet and a cross-sectional analysis along to the yellow line. (d) SEM image of a1Ymicrosheet (scale bar, 10 μm). (e) Schematic representation of the multilamellar structure of1Y. Aromatic, aliphatic and hydrophilic sublayers are indicated by orange, green and yellow, respectively. (f) Schematic representation of in-plane oblique packing of1in1Y. The yellow plates correspond to two molecules of1. Figure 5: Analysis of packing structures of 1Y . ( a ) PXRD patterns of 1Y with major d -spacings in Å. Small diffractions derived from the in-plane molecular ordering are indicated by black triangles. Inset (surrounded by red dotted square): Schematic representation for the experimental setup of transmission mode 2D-WAXD of 1Y microsheets deposited on 0.03-mm thickness glass substrate using synchrotron radiation and the observed diffraction profile. ( b ) AFM image of the surface of 1Y microsheet and a cross-sectional analysis along to the yellow line. ( c ) AFM image of the surface of 1Y microsheet and a cross-sectional analysis along to the yellow line. ( d ) SEM image of a 1Y microsheet (scale bar, 10 μm). ( e ) Schematic representation of the multilamellar structure of 1Y . Aromatic, aliphatic and hydrophilic sublayers are indicated by orange, green and yellow, respectively. ( f ) Schematic representation of in-plane oblique packing of 1 in 1Y . The yellow plates correspond to two molecules of 1 . Full size image The in-plane molecular ordering in the 1Y microsheet was further revealed by two-dimensional (2D) wide-angle X-ray diffraction (WAXD) analysis. AFM ( Fig. 5c ) and scanning electron microscopy (SEM; Fig. 5d ) images showed that the microsheets of 1Y have thicknesses of 100–250 nm and were formed in the face-on arrangement on the glass substrate. Transmission mode 2D WAXD analysis using the X-ray beam perpendicular to the microsheets showed diffractions corresponding to d -spacings of 11.6, 5.92, 5.09, 4.57 and 3.95 Å (inset in Fig. 5a ). These diffractions were assigned to an oblique lattice with lattice parameters a =11.6 Å, b =5.09 Å and γ=94° ( Fig. 5f ). The short lattice parameter b indicates the presence of cofacially π–π-stacked π-conjugated moieties. In contrast, the PXRD patterns of 1O were fairly simple and were attributed to a lamellar mesophase with a 34.2-Å interlayer spacing ( Fig. 6a ). The absence of reflections for in-plane ordering may reflect the dynamic nature of the individual molecules in this phase; the π-conjugated chromophores were rotating around their long molecular axis. When 1O was thermally generated on a glass substrate via slow cooling of the isotropic melt, a four-brush schlieren texture was observed by POM ( Fig. 6b ). For thinner 1O samples prepared by sandwiching two glass substrates, a focal-conic fan texture was observed with extinction brushes that were inclined by 45° with respect to the crossed polarizers ( Fig. 6c ). These POM textures are typical of smectic C liquid crystalline mesophases with homeotropic (schlieren) and planar orientations (focal-conic fan). The 2D WAXD pattern of sheared 1O showed no diffraction peaks in the small-angle region, suggesting the absence of in-plane molecular ordering. 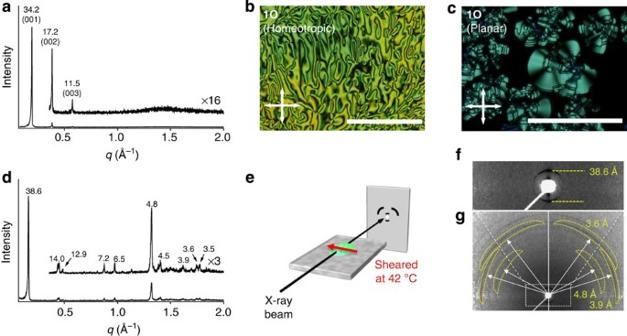Figure 6: Analysis of packing structures of1Oand1G. (a) PXRD pattern of1O. (b,c) Polarized optical micrographs of homeotropically oriented1Oon a glass substrate (b, scale bar, 100 μm) and planarly oriented1Obetween two glass substrates (c, scale bar, 20 μm). The samples were prepared via thermal procedure. Arrows indicate the direction of polarizer and analyser. (d) PXRD pattern of1G. (e) Schematic representation for the experimental setup of in-plane 2D PXRD measurements of1Gsheared at 42 °C along to the red arrow. (f,g) 2D diffraction pattern of the sheared1Gin small-angle (f) and wide-angle region (g). Forg, broad diffractions were surrounded by yellow dotted lines. Figure 6: Analysis of packing structures of 1O and 1G . ( a ) PXRD pattern of 1O . ( b , c ) Polarized optical micrographs of homeotropically oriented 1O on a glass substrate ( b , scale bar, 100 μm) and planarly oriented 1O between two glass substrates ( c , scale bar, 20 μm). The samples were prepared via thermal procedure. Arrows indicate the direction of polarizer and analyser. ( d ) PXRD pattern of 1G . ( e ) Schematic representation for the experimental setup of in-plane 2D PXRD measurements of 1G sheared at 42 °C along to the red arrow. ( f , g ) 2D diffraction pattern of the sheared 1G in small-angle ( f ) and wide-angle region ( g ). For g , broad diffractions were surrounded by yellow dotted lines. Full size image The crystalline phase 1G exhibited the most complicated diffraction pattern that contained an intense diffraction at 38.6 Å and a number of weak diffractions indicative of crystallization-induced, 3D molecular order ( Fig. 6d ). We found that this crystalline phase became waxy when heated in the range of 40–50 °C, whereas the emission colour remained green. This behaviour is possibly because of the melting of the TEG sublayers that can be used to orient the molecules mechanically. Therefore, we performed an in-plane, 2D PXRD measurement of a thin-film sample of 1G sheared on a glass substrate at 42 °C ( Fig. 6e ). On the meridian, a diffraction corresponding to the interlayer distance was observed ( Fig. 6f ), which suggested that the basic lamellar structure would be preserved upon crystallization of 1O to 1G . In the wide-angle region, broad diffractions were observed at 4.8, 3.9 and 3.6 Å; the centres of these diffraction peaks were not located on the meridian ( Fig. 6g ). Although a clear assignment of the diffraction pattern could not be made, these observations suggest that the inclination of the molecules within the layers is also preserved upon crystallization of 1O . The parent compound 1 did not form crystals suitable for X-ray crystallography; however, we obtained structural insight into the mesomorphic 1O from a single-crystal structural analysis of a reference compound ( 2 ) that lacked amphiphilic side chains ( Supplementary Data 1 ). Compound 2 yielded plate-like single crystals from an ethyl acetate solution that exhibited an orange emission ( Supplementary Fig. 5a ). Because the emission spectrum of crystal 2 is very similar to that of 1O ( Fig. 7a ), the crystal structural analysis of 2 revealed the packing state of the π-conjugated core in the mesomorphic phase 1O . The crystal structure of 2 has a triclinic space group P -1 and is characterized by a lamellar ordering of an inclined molecular packing ( Supplementary Fig. 5b ). The dipolar molecules are packed within single layers in the antiparallel arrangement because of the absence of amphiphilicity. When the lamellar structure is viewed from the direction of the molecular long axis, a herringbone arrangement of the π-conjugated planes is revealed ( Fig. 7b ). The π-conjugated planes between the neighbouring herringbone rows have a dihedral angle of 40.4°, suggesting the absence of π–π stacking interactions. This finding indicates that the orange emission is derived from the oligo( p -phenylenevinylene) luminophores with no apparent overlap of their π-planes. More importantly, the oligo( p -phenylenevinylene) cores alternately adopt chair-like or boat-like conformations from row to row ( Fig. 7b ). Whereas the chair-like conformer is ordered, the boat-like conformer is disordered because of the adoption of two crystallographically independent conformations with different occupancies (I:II=41:59; Fig. 7c ) [28] . The temperature-dependent crystallographic analyses performed at temperatures from −150 to 20 °C did not show a change in the occupancies of the two boat-like conformers, which suggests that they are not dynamically interconverted in the crystal. Nevertheless, the boat-like conformers I and II exhibit a geometrical distortion: the two C–C bonds linking the central phenylene unit and the vinylene groups show an angle ( θ ) of 161° and 167°, respectively, which deviate from linearity compared with the nearly linear shape of the chair-like conformer ( θ =178°; Fig. 7d ). This geometrical distortion must be responsible for the long-wavelength emission because of intramolecular charge–transfer interactions. 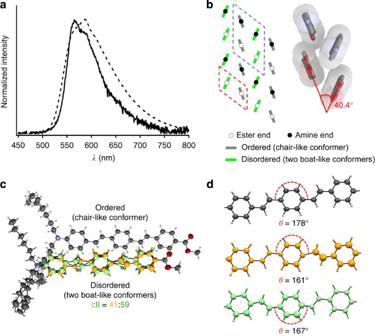Figure 7: X-ray crystallographic study of2. (a) Fluorescence spectra (λex=400 nm) of2(solid line) and1O(dashed line). (b) Left: schematic representation of the herringbone arrangement of the oligo(p-phenylenevinylene) π-conjugated unit by viewing from the direction along to the long molecular axis. Grey and green bars indicate the ordered and disordered π-conjugated units, respectively. Open and closed circles indicate the ester and amine end of the π-conjugated units, respectively. Right: the molecular packing of a tetrameric unit extracted from the crystal structure (surrounded by blue dotted lines). (c) ORTEP drawing of a dimeric unit (surrounded by red dotted lines inb) composed of the crystallographically ordered π-conjugated unit with a chair-like conformation (grey) and crystallographycally disordered π-conjugated units with two boat-like conformations. Conformers I and II are coloured with yellow and green, respectively. Occupancies of the conformers I and II are 41% and 59%, respectively. (d) Comparison of the distortion of π-conjugated systems in the three conformers. Figure 7: X-ray crystallographic study of 2 . ( a ) Fluorescence spectra ( λ ex =400 nm) of 2 (solid line) and 1O (dashed line). ( b ) Left: schematic representation of the herringbone arrangement of the oligo( p -phenylenevinylene) π-conjugated unit by viewing from the direction along to the long molecular axis. Grey and green bars indicate the ordered and disordered π-conjugated units, respectively. Open and closed circles indicate the ester and amine end of the π-conjugated units, respectively. Right: the molecular packing of a tetrameric unit extracted from the crystal structure (surrounded by blue dotted lines). ( c ) ORTEP drawing of a dimeric unit (surrounded by red dotted lines in b ) composed of the crystallographically ordered π-conjugated unit with a chair-like conformation (grey) and crystallographycally disordered π-conjugated units with two boat-like conformations. Conformers I and II are coloured with yellow and green, respectively. Occupancies of the conformers I and II are 41% and 59%, respectively. ( d ) Comparison of the distortion of π-conjugated systems in the three conformers. Full size image Optical properties Solid-state absorption measurements revealed that only 1Y featured a strong exciton interaction between the π-conjugated luminophores (left axis; Fig. 8a ). A solution of monomeric 1 in acetonitrile exhibited an intense absorption band at 412 nm. After the solution was cast to form 1Y films, a large hypsochromic shift to 333 nm was observed. According to the exciton theory [29] , this spectral change is indicative of π-conjugated chromophores stacked face-to-face (H-type aggregation). When 1Y was converted to 1O by gentle pressing, the absorption band at 390 nm increased, reaching almost the same intensity as the hypsochromically shifted band and clearly demonstrating a decrease in the electronic interactions between the π-conjugated chromophores in the mesomorphic state. The spectrum of 1G resembled that of 1O but was more vibronically structured to reflect the rigid molecular packing in this phase. These absorption features, combined with the DSC and PXRD results, demonstrate that the mechanochromic luminescence from 1Y to 1O was caused by the loss of excitonic interactions between the dipolar π-conjugated systems, whereas that from 1O to 1G was caused by the increased rigidity of the molecular structure due to crystallization. 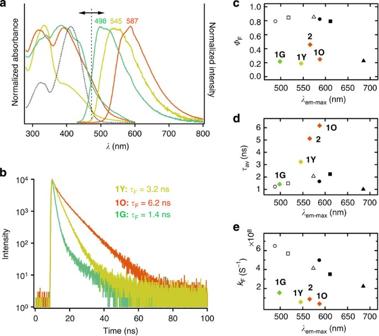Figure 8: Absorption and fluorescence properties of1. (a) UV/Vis absorption (left axis) and fluorescence spectra (right axis,λex=400 nm) of1Y,1Oand1G. The dotted curve represents the UV/Vis spectrum of the acetonitrile solution (c=1.0 × 10−5M). (b) Fluorescence decay profiles of1Y,1Oand1Gwith their fluorescence lifetimes (τF). (c–e) Scatter plot of fluorescence quantum yield (c), average fluorescence lifetime (d) and radiative rate constant (e) of1G,1Y,1O, single crystal of2and solutions of1(open circles, hexane; open squares, toluene; open triangles, chloroform; closed circles, tetrahydrofuran; closed squares, dichloromethane; and closed triangles, acetonitrile). Figure 8: Absorption and fluorescence properties of 1 . ( a ) UV/Vis absorption (left axis) and fluorescence spectra (right axis, λ ex =400 nm) of 1Y , 1O and 1G . The dotted curve represents the UV/Vis spectrum of the acetonitrile solution ( c =1.0 × 10 −5 M). ( b ) Fluorescence decay profiles of 1Y , 1O and 1G with their fluorescence lifetimes ( τ F ). ( c – e ) Scatter plot of fluorescence quantum yield ( c ), average fluorescence lifetime ( d ) and radiative rate constant ( e ) of 1G , 1Y , 1O , single crystal of 2 and solutions of 1 (open circles, hexane; open squares, toluene; open triangles, chloroform; closed circles, tetrahydrofuran; closed squares, dichloromethane; and closed triangles, acetonitrile). Full size image The emission properties of the three distinct phases were studied via steady-state (right axis; Fig. 8a ) and time-resolved fluorescence spectroscopy ( Fig. 8b ), and the fluorescence quantum yield ( Φ F ), average fluorescence lifetime ( τ av ) and radiative rate constant ( k F ) are summarized in Supplementary Table 2 . We also measured the fluorescence properties of 1 dissolved in various solvents with different polarities ( Supplementary Table 1 ), and compared the values with those of the solid phase by plotting the results against the emission maxima ( Fig. 8c–e ). All the solid phases displayed smaller Φ F ( Fig. 8c ) and k F ( Fig. 8e ) values compared with those in the solution phases; these smaller values can be attributed to possible energy transfer in the bulk materials. In contrast to the nearly λ em-max -independence of τ av (1–2 ns) in the solution phases, the τ av of the solid phases exhibited a large dependence on λ em-max ( Fig. 8d ). This observation suggests that the geometrical freedom and/or intermolecular interaction of luminophores are responsible for the emission wavelength in the solid states. The H-aggregated phase 1Y had a maximum emission at 545 nm with a 3.24-ns lifetime and a radiative rate constant of 5.9 × 10 7 s –1 . In general, H-type aggregation causes strong fluorescence quenching, as is typically observed for dipolar merocyanine dyes [30] , [31] . If the largest Stokes shift (11,681 cm –1 ) among the three phases is taken into consideration, the fluorescence from 1Y could arise from an imperfect H-type stacking with a rotational displacement around the stacking axis, thereby allowing the radiative decay to originate from the lower-lying exciton state [32] . The mesomorphic phase 1O exhibited a more red-shifted emission that reached a maximum at 587 nm (Stokes shift=8,539 cm –1 ) and was unchanged after transformation into isotropic phase Iso . The longest τ av ( Fig. 8d ) but the same approximately k F value as that of 1Y ( Fig. 8e ) indicates that the intermolecular energy transfer was suppressed in 1O compared with in 1Y because of the absence of the excitonic interaction between the luminophores. Importantly, the crystal of 2 involving distorted π-conjugated moieties exhibited an orange fluorescence with emission properties analogous to those of 1O ( Fig. 8d,e ), except for a higher Φ F (0.46; Fig. 8c ). Therefore, similar geometric distortion of the π-conjugated systems occurs in this fluid phase’s excited state, which may facilitate intramolecular charge–transfer interactions to generate a relatively long-lived, red-shifted emission. In contrast, the crystalline phase 1G exhibited an emission maximum at the shortest wavelength (498 nm) with the smallest Stokes shift (6,090 cm –1 ) and the shortest τ av (1.42 ns) among the three phases. These emission properties are analogous to those of the toluene solution ( Fig. 8d ): the polar excited state was weakly stabilized by the solvent. Therefore, the bluish-green emission from 1G could be derived from monomeric luminophores packed in a rigid crystalline phase. Although 1G # and 1G exhibited almost identical absorption spectra ( Supplementary Fig. 4 ), 1G # had an emission maximum at 547 nm, similar to that of 1Y ( Supplementary Fig. 6 ). Therefore, an energy transfer may occur from the excited state of the monomeric ( 1G ) to the π–π stacked chromophores ( 1Y ) present in small quantities [33] . Controlling crystallization using a lithium salt The mechanically induced phase conversion from 1O to 1G # (that is, the less crystalline form of 1G ) was found to be caused by the nucleation and propagation of a crystalline phase in a mesomorphic state [34] . After an edge of the 1O sample was rubbed on a glass substrate, the crystallization developed toward the surrounding area at ~1.0 mm h –1 at room temperature (panels a,b in Fig. 9A ). The same phase transformation was triggered by touching a small ‘seed’ of 1G # to 1O (see Supplementary Movies 2 and 3 ), similar to crystal growth in solution. The phase conversion could be halted by heating the sample to 50 °C; this temperature is higher than the isotropization temperature ( T iso ) of 1O (47 °C) but lower than that of 1G (54 °C; panels c,d). The process was restarted when the sample was cooled to r.t. (panels e,f). Therefore, the phase conversion does not transmit to Iso . On the basis of these observations, we conclude that subjecting the metastable 1O to strong mechanical stimulation generates a small nucleus of thermodynamically stable 1G # that partially consists of π–π-stacked luminophores similar to 1Y . The 1G # region could then spontaneously propagate. Thermal annealing of 1G # below its isotropization temperature ( T iso =54 °C) induces another structural rearrangement to yield 1G , freeing all of the luminophores from the π–π stacking interactions. 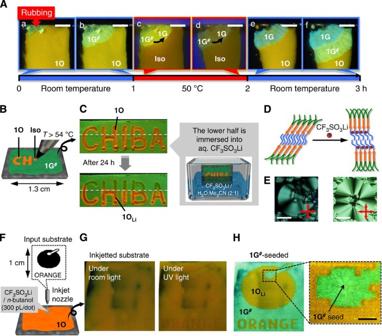Figure 9: Rubbing and seeding induced phase transition of1Oto1G. (A) Photographs revealing the spontaneous propagation of1G#on1Ounder UV light. (a,b) Propagation at r.t. ; (c,d) propagation paused at 50 °C; (e,f) propagation restarted at r.t. Scale bars, 1 mm. (B) Schematic representation of thermal writing usingIso(converted to1Oupon cooling) generated with a soldering pen on1G#. (C) Photographs exhibiting the control over the auto-erasure of1Oon1G#under UV light. Only the lower half of the glass plate was immersed in an aqueous acetonitrile solution containing CF3SO3Li. (D) Schematic representation of orientational change of1upon complexing with the lithium salt (shown by red balls). (E) POM images of1O(left, scale bar, 10 μm) and1OLi(right, scale bar, 50 μm). Red arrows indicate the direction of polarizer and analyser. (F) Schematic representation of inkjet writing of a cartoon picture of an orange fruit and the characters ‘ORANGE’ (~1 cm in size) on1Oby usingn-butanol solution of CF3SO3Li (5 wt%). (G) Photographs of the inkjetted sample under room light (left) and under UV light (right). (H) Photograph of the inkjetted sample under UV light after1G#seeding. Inset shows the fluorescent microscopic image of a part of the orange picture (scale bar, 0.5 mm). Figure 9: Rubbing and seeding induced phase transition of 1O to 1G . ( A ) Photographs revealing the spontaneous propagation of 1G # on 1O under UV light. (a,b) Propagation at r.t. ; (c,d) propagation paused at 50 °C; (e,f) propagation restarted at r.t. Scale bars, 1 mm. ( B ) Schematic representation of thermal writing using Iso (converted to 1O upon cooling) generated with a soldering pen on 1G # . ( C ) Photographs exhibiting the control over the auto-erasure of 1O on 1G # under UV light. Only the lower half of the glass plate was immersed in an aqueous acetonitrile solution containing CF 3 SO 3 Li. ( D ) Schematic representation of orientational change of 1 upon complexing with the lithium salt (shown by red balls). ( E ) POM images of 1O (left, scale bar, 10 μm) and 1O Li (right, scale bar, 50 μm). Red arrows indicate the direction of polarizer and analyser. ( F ) Schematic representation of inkjet writing of a cartoon picture of an orange fruit and the characters ‘ORANGE’ (~1 cm in size) on 1O by using n -butanol solution of CF 3 SO 3 Li (5 wt%). ( G ) Photographs of the inkjetted sample under room light (left) and under UV light (right). ( H ) Photograph of the inkjetted sample under UV light after 1G # seeding. Inset shows the fluorescent microscopic image of a part of the orange picture (scale bar, 0.5 mm). Full size image Because of the ‘seeding’ effect of 1G # on 1O , thermal writing created by a soldering iron ( Fig. 9B ) on the mechanically developed 1G # film (>54 °C) was automatically erased while the sample was maintained at r.t. for 1 h (the upper half of the characters ‘CHIBA’ in Fig. 9C ). The volatility of the thermal writing on 1G # could be controlled by treating the substrate with aqueous solutions of a lithium salt. When the lower half of a sample containing the characters ‘CHIBA’ thermally written on 1G # was immersed into an aqueous CF 3 SO 3 Li solution (~10 wt%) for a few seconds, the immersed portion of the characters continued to exhibit orange emission with almost the same fluorescence colours (the lower half of the characters ‘CHIBA’ in Fig. 9C ). The PXRD analysis revealed that 1O was converted to 1O Li ( T iso =120 °C) by forming chelation complexes in the TEG moieties ( Supplementary Fig. 7 ) [35] , [36] . The interlayer distance was extended from 34.2 Å in 1O to 60.1 Å in 1O Li ; this change could be ascribed to the cancellation of the molecular tilt owing to the loss of the interdigitation of the TEG moieties upon chelation with the salt ( Fig. 9D ). The cancellation of the molecular tilt was further supported by the focal-conic fan texture of 1O Li , which exhibited extinction brushes parallel to the polarizers ( Fig. 9E ). The inflexibility of the luminophore caused by the Li chelation and a less tilted structure in 1O Li are responsible for the higher T iso of 1O Li . The phase-transition property of 1O , which was controllable through the treatment with the lithium salt, was used in invisible inkjet imaging, which can be decoded by a ‘molecular key’ that can induce a selective phase change on 1O . We prepared thin films of 1O and created invisible images of a cartoon picture of an orange fruit and the characters ‘ORANGE’ on the film via inkjet printing (300 pL per dot) with an n -butanol solution of CF 3 SO 3 Li (5 wt%; Fig. 9F ). The printed image was not clearly discernible under room light or even under UV illumination ( Fig. 9G ) because the resulting 1O Li has emission maximum identical to that of 1O . However, when small crystallites of 1G # were seeded onto several parts of the film, only the background 1O was converted into 1G # after several hours. In contrast, the 1O Li in the imaged area remained unchanged, thereby revealing the printed images as orange emissions on the green-emitting background under UV illumination ( Fig. 9H ). Fluorescence microscopy observations revealed that the diffusion of the lithium salt on 1O was suppressed within ~30 μm (magnified image in Fig. 9H ), which ensures a high resolution for imaging on the micrometre scale. Because the use of an aqueous solution of CF 3 SO 3 Li resulted in more unambiguous images ( Supplementary Fig. 8 ), the selection of the solvent system for the inkjet procedure is important to minimize the diffusion of the salt within the mesophase. We have demonstrated that dipolar π-conjugated systems with proper amphiphilicity can form several metastable self-assembled phases with distinct packing states of the π-conjugated units and emission properties. The designed metastable state is converted into a more stable packing state via the application of both weak ( 1Y to 1O ) and strong ( 1O to 1G # ) mechanical stimuli ( Fig. 1c ). A mechanism for the mechano-induced phase conversion from 1Y to 1O can be explained as follows: the evaporation of the acetonitrile solution containing 1 forms a metastable, multilamellar organized structure ( 1Y ); this process is driven by the segregation of incompatible molecular components. The aggregation facilitates face-to-face π–π stacking interactions between the dipolar π-conjugated systems to generate the yellow emission. Because of the energetically unfavourable parallel orientation of the dipole moments, a weak mechanical stimulus can easily convert this metastable, aggregated state into a mesomorphic state ( 1O ). The similarity between the emission properties of 1O and the single crystal of 2 demonstrates that the dipolar π-conjugated systems are dynamically twisted in the mesomorphic state within the layers. The twisted π-conjugated system can induce intramolecular charge transfer, thus resulting in emission in the longest-wavelength region. Although the dipolar repulsion between stacked π-conjugated systems in 1Y should be considerably dissolved by the transition into 1O , it must still remain in this fluidal mesophase where π-conjugated systems can freely rotate within π-conjugated sublayers. Furthermore, the packing density mismatch between the π-conjugated sublayers and the interdigitated TEG sublayers as well as the Gemini-shaped aliphatic sublayers should make this phase thermodynamically unstable. This metastability facilitates crystallization to 1G # through mechanical stimulus or seeding to yield the green emission derived from the planar π-conjugated systems that are free of π–π stacking interactions. The lithium salt adjusts the volume of the three incompatible molecular components of 1 by being sandwiched between the TEG chains of neighbouring parallel-oriented molecules, which stabilizes the mesophase against crystallization ( Fig. 9D ). We can apply this lithium-responsive property of 1O to invisible inkjet printing, which is subsequently revealed using a small crystal of the same material as a ‘molecular key’. In conclusion, we demonstrate that dipolar π-conjugated systems with proper amphiphilicity can form several metastable self-assembled phases with distinct molecular packing and emission properties. The designed metastable state is converted into a more stable packing state by the application of both weak and strong mechanical stimuli. The rationale for this behaviour involves the unfavourable parallel orientation of the molecular dipole moments that become kinetically trapped upon segregation between incompatible molecular regions. The present study provides a basic molecular strategy for the design of new mechano-responsive compounds with various π-conjugated luminophores. Materials Compounds 1 and 2 were synthesized according to Supplementary Fig. 9 based on the synthetic methods reported previously [37] . All starting materials and reagents were purchased from commercial suppliers and used as received. 1 H NMR ( Supplementary Figs 10 and 12 ) and 13 C NMR ( Supplementary Figs 11 and 13 ) and HRMS ( Supplementary Figs 14 and 15 ) of 1 and 2 were included in the Supplementary Methods . Measurements The solvents for the spectroscopic measurements were all spectral grade and used without further purification. Solid-state UV/Vis absorption spectra were recorded on a JASCO V660 spectrophotometer. Fluorescence spectra were recorded on a JASCO FP6600 spectrofluorometer and a Hitachi F-7000 spectrometer. Fluorescence microscopic spectrum of the crystal of 2 was recorded on a photonic multichannel analyser (Hamamatsu Photonics). 13 C- and 1 H-NMR spectra were recorded on Bruker DPS300, JEOL JNM-ECS400 and JEOL JNM-ECA500 spectrometers and chemical shifts are reported in p.p.m. ( δ ) with the signal of tetramethylsilane (TMS) as internal standard. electrospray ionization (ESI)- and atmospheric pressure chemical ionization-high-resolution mass spectrometry (ACPI-HRMS) were measured on a Exactive (Thermo Scientific). Elemental analyses were performed at Chemical Analysis Center in Chiba University. Fluorescence quantum yields were measured on Absolute PL Quantum Yield Measurement System C9920-02 (Hamamatsu Photonics). Emission lifetime measurements were recorded on Quantaurus-Tau spectrometers (Hamamatsu Photonics). DSC was performed on SII DSC6220. Heating and cooling rate is 2 °C min −1 . Polarized OM observation was carried out using an Olympus BX51 OM system with a Linkam temperature-controlled heating stage. SEM observation was acquired by using JEOL JSM-6330F SEM. AFM observation was carried out using Nanoscope Multimode 8 (Bruker AXS). PXRD analysis was carried out with a Rigaku Rint-2200 X-ray diffractometer with monochromated CuKα 1 ( λ =1.54 Å) radiation and temperature-controlled heating stage. 2D WAXD measurements were performed with synchrotron radiation ( λ =0.75 Å) at BL02B2 in SPring-8 with the approval of Japan Synchrotron Radiation Research Institute (JASRI). The samples were prepared on a glass substrate (thickness=0.03 mm). In-plane X-ray diffraction In-plane X-ray diffraction of sheared 1G film was carried out with TRY-DXGSA-HHIP vertical X-ray diffractometer (TRY SE Co., Ltd) equipped with an imaging plate holder and a hot stage parallel to the glass plate. The sample sheared on a glass plate (glass thickness: 0.05 mm) was irradiated by monochromated CuKα 1 X-ray ( λ =1.54 Å, beam diameter: 0.5 mm; voltage: 40 kV; current: 30 mA; and camera length: 138 mm). The diffraction was recorded on an imaging plate (200 mm × 200 mm), and the image was read by an FLA-7000 imaging plate reader (Fujifilm Co., Ltd). Single-crystal X-ray analysis Measurements of the single crystal of 2 were performed on a Rigaku R-AXIS RAPID diffractometer equipped with a graphite-monochromated Mo-Kα radiation source. The diffraction data were collected at various temperatures and the crystallographic parameters are summarized in Supplementary Table 3 . The structure was determined using direct methods and was expanded using Fourier techniques. Non-hydrogen atoms were refined anisotropically, except in the case of the disordered oligo( p -phenylenevinylene) cores. Hydrogen atoms were refined using the riding model. All the calculations were performed using the CrystalStructure crystallographic software package, except for refinement, which was performed using the SHELXL-97 software programme. Inkjet printing Inkjet printing experiments were performed using a LaboJet-500 inkjet printer, Microjet Corporation, Japan. An n -butanol solution of CF 3 SO 3 Li (5 wt%) was dotted (300 pL per dot) onto thin films of 1O to draw invisible images. After the inkjet printing, small crystallites of 1G # were seeded onto the film. After the sample was maintained at r.t. for 3 h, the background 1O was fully converted to 1G # to reveal the invisible images. How to cite this article: Yagai, S. et al . Design amphiphilic dipolar π-systems for stimuli-responsive luminescent materials using metastable states. Nat. Commun. 5:4013 doi: 10.1038/ncomms5013 (2014). Accession codes: The X-ray crystallographic coordinate for 2 reported in this article have been deposited at the Cambridge Crystallographic Data Centre (CCDC) under deposition numbers CCDC 986425. These data can be obtained free of charge from The Cambridge Crystallographic Data Centre via www.ccdc.cam.ac.uk/data_request/cif .